Fundamental rate-loss tradeoff for optical quantum key distribution Since 1984, various optical quantum key distribution (QKD) protocols have been proposed and examined. In all of them, the rate of secret key generation decays exponentially with distance. A natural and fundamental question is then whether there are yet-to-be discovered optical QKD protocols (without quantum repeaters) that could circumvent this rate-distance tradeoff. This paper provides a major step towards answering this question. Here we show that the secret key agreement capacity of a lossy and noisy optical channel assisted by unlimited two-way public classical communication is limited by an upper bound that is solely a function of the channel loss, regardless of how much optical power the protocol may use. Our result has major implications for understanding the secret key agreement capacity of optical channels—a long-standing open problem in optical quantum information theory—and strongly suggests a real need for quantum repeaters to perform QKD at high rates over long distances. The goal of quantum key distribution (QKD) is to generate a shared secret key between two distant parties Alice and Bob, such that the key is perfectly secret from any eavesdropper, Eve. Since the invention of the BB84 protocol [1] , the theory and practice of QKD has come a long way. Various different QKD protocols have been proposed in the last three decades [2] , some of which are now turning from science into practical technologies [3] , [4] , [5] . Security of QKD has now been proven for many protocols and under practical limitations such as a finite key length [6] , [7] . It is well recognized that the key rates of all known QKD protocols (such as BB84 (ref. 1 ), E91 (ref. 8 ) and CV-GG02 (ref. 9 )) decay exponentially with distance. To obtain a large key rate across a long-distance link, the link can be divided into many low-loss segments separated by trusted (physically secured) relay nodes. Interestingly, however, quantum mechanics permits building QKD protocols using devices called quantum repeaters, which if supplied at the relay nodes, would make it unnecessary to physically secure them, thus enabling long-distance high-rate QKD. Quantum repeater technology, in particular the ones built using quantum memories, has been a subject of intense investigation in recent years [10] , [11] ; however, an operational demonstration of a quantum repeater has proven extremely challenging and is yet to be conducted (note that some repeater protocols without quantum memory have been proposed recently [12] , [13] ; however, their implementation is still challenging). The natural question that thus arises is whether there are yet-to-be-discovered optical QKD protocols that could circumvent the exponential rate-distance tradeoff of BB84 and transmit at high rates over long distances without the need for quantum repeaters. In this paper, we establish that it is not possible to do so. We employ information-theoretic techniques in order to establish our main result. The secret key agreement capacity of a quantum channel is the highest rate (bits per channel use) at which a shared key can be reliably and securely generated using the channel many times in conjunction with unlimited two-way classical communication over an authenticated public channel. This paper establishes that, regardless of the QKD protocol used, a fundamental limit on the secret key agreement capacity of a lossy optical channel is given by an upper bound that is solely a function of the channel loss, that is, independent of the transmit power. We show that the bound is nearly optimal at high loss, the regime relevant for practical QKD. We also compare our upper bound and the best-known achievable rate with the ideal BB84 and CV-GG02 protocols. We find that even though there is room for improvement over these protocols, there is essentially no gap in the rate-loss scaling. We thereby place on a firm foundation the need for quantum repeaters for high-rate QKD over long distances with no trusted relays. We note that the upper bound proved here is a so-called ‘weak converse’ upper bound, meaning that if the communication rate of any secret key agreement protocol exceeds this bound, then our theorem implies that its reliability and security can never be perfect, even in the asymptotic limit of many channel uses (we will also discuss the issue of a finite number of channel uses below and in the Methods section). A generic point-to-point QKD protocol is illustrated in Fig. 1 . In the protocol, the sender Alice transmits over n independent uses of the quantum channel . The legitimate receiver Bob obtains the outputs of the channel uses. Note that Alice could send product or entangled states. They are also allowed unlimited two-way public classical communication over an authenticated channel, in order to generate shared secret key. The adversary Eve is assumed to be ‘all-powerful’: one who has access to the full environment of the Alice-to-Bob quantum channel, the ‘maximal’ quantum system to which she can have access. Optically, this translates to Eve being able to collect every single photon that does not enter Bob’s receiver. Eve may also actively attack, for instance by injecting a quantum state into the channel. She has access to all the public classical communications between Alice and Bob. Finally, Eve is assumed to be able to store the quantum states she obtains over all n channel uses without any loss or degradation, and she can make any collective quantum measurement on those systems, in an attempt to learn the secret key. In the theory of QKD, one attributes all channel impairments (such as loss, noise, turbulence and detector imperfections) collectively measured by Alice and Bob during a channel-estimation step of the protocol, to adversarial actions of the worst case Eve, with which the measured channel is ‘consistent’ (even though in reality all those impairments may have been caused by non-adversarial natural phenomena). Alice and Bob then run a key generation protocol aiming to generate the secret key at a rate close to the secret key agreement capacity of that channel. It is hard in general to calculate this capacity precisely, and even more so to come up with protocols that can attain the key rates close to that capacity. 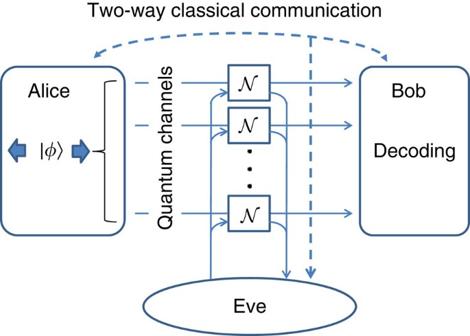Figure 1: A generic point-to-point QKD protocol. Alice transmits quantum state vianforward uses of a quantum channel to Bob. They are also allowed to use unlimited forward and backward public classical communications over an authenticated classical channel. Figure 1: A generic point-to-point QKD protocol. Alice transmits quantum state via n forward uses of a quantum channel to Bob. They are also allowed to use unlimited forward and backward public classical communications over an authenticated classical channel. Full size image In this paper, we show a strong limitation on the secret key agreement capacity of a general memoryless quantum channel. More precisely, we provide a simple upper bound on the two-way assisted private capacity P 2 ( ) of a quantum channel . Note that the capacity for the secret key agreement using QKD as discussed above is equal to the capacity for private communication with unlimited public discussion because of the one-time pad protocol. We first define a new quantity, the squashed entanglement of a quantum channel, and show that it is a simple upper bound on P 2 ( ) for any quantum channel . We then apply it to the pure-loss optical channel η with transmittance η ε[0,1]. Channel loss is an important and measurable impairment both for free space and fibre optical links, and is directly tied to the communication distance (for example, a low-loss fibre may have a loss of 0.2 dB km −1 ). Since any excess noise in the channel or detectors can only reduce the extractable key rate, our upper bound on P 2 ( η ) imposes a fundamental upper limit on the secret key rate of any point-to-point QKD protocol over a lossy optical channel not assisted by any quantum repeater. We will establish the following upper bound: In the practical regime of high loss ( η ≪ 1), we will argue that this upper bound is only a factor of two higher than the best-known lower bound, P 2 ( η )≥log(1/(1− η )) (ref. 14 ). We will also extend our upper bound to the more general scenario of QKD using a two-way quantum channel with unlimited public discussion, which was discussed recently in ref. 15 . Finally, we will compare our upper bound and the best-known lower bound to the rate achievable by the BB84 and the CV-GG02 protocols under best-case operating conditions as well as compare with the performance of these protocols under realistic operating conditions. Squashed entanglement Before discussing our main results, we briefly review the squashed entanglement, which plays an important role in our work. The secret key agreement capacity assisted by public communication was defined for a classical channel p Y , Z | X ( X =Alice, Y =Bob, Z =Eve), independently by Maurer [16] , and Ahlswede and Csiszár [17] , who proved lower and upper bounds on the capacity. Maurer and Wolf [18] later introduced the intrinsic information I ( X ; Y ↓ Z )≡min{ I ( X ; Y | Z ′): P X , Y , Z , Z ′ = P X , Y , Z P Z ′| Z }, and proved that this quantity optimized over all channel input distributions is a sharp upper bound on the secret key agreement capacity of p Y , Z | X . Leveraging strong parallels discovered between secrecy and quantum coherence [19] , [20] , [21] , Christandl and Winter [22] extended the intrinsic information quantity to the realm of quantum information theory. They defined the squashed entanglement E sq ( A ; B ) ρ of a bipartite quantum state ρ AB and proved it to be an upper bound on the rate at which two parties can distil maximally entangled (Bell) states from many copies of ρ AB using local operations and classical communication (LOCC). Using a similar technique, the squashed entanglement was proved to upper bound the distillable secret key rate [23] , [24] . The squashed entanglement of a bipartite state ρ AB is defined as where I ( A ; B | E ′)≡ H ( AE ′)+ H ( BE ′)− H ( E ′)− H ( ABE ′) is the conditional quantum mutual information and the infimum is taken over all noisy ‘squashing channels’ E → E ′ taking the system E of a purification | φ ρ › ABE of ρ AB to a system E ′ of arbitrary dimension. In related work, Tucci [25] , [26] has defined a functional bearing some similarities to squashed entanglement. We can interpret E sq ( A ; B ) ρ as quantifying the minimum remnant quantum correlations between A and B after an adversary possessing the purifying system E performs a quantum operation on it with the intent of ‘squashing down’ the correlations that A and B share. It should also be noted that among the many entanglement measures, squashed entanglement is the only one known to satisfy all eight desirable properties that have arisen in the axiomatization of entanglement theory [22] , [27] , [28] , [29] . Squashed entanglement of a quantum channel The upper bound from ref. 23 on the distillable key rate applies to the scenario in which Alice and Bob share many copies of some bipartite state ρ AB . In order to upper bound the key agreement capacity of a channel, we define the squashed entanglement of a quantum channel A ′→ B as the maximum squashed entanglement that can be registered between a sender and a receiver with access to the input A ′ and output B of this channel, respectively: where ρ ≡ ρ AB ≡ A ′→ B (| φ ›‹ φ | AA ′ ). Note that, in the above formula, we can take a maximum rather than a supremum if the input space is finite-dimensional because, in this case, the input space is compact and the squashed entanglement measure is continuous [28] . In addition, we can restrict the optimization to be taken over pure bipartite states because of the convexity of squashed entanglement [22] . We now prove that E sq ( ) plays an operational role analogous to intrinsic information, that is, it upper bounds the secret key agreement capacity P 2 ( ). Theorem 1: E sq ( ) is an upper bound on P 2 ( ), the private capacity of assisted by unlimited forward and backward classical communications: Proof: first recall that the squashed entanglement is a secrecy monotone, that is, it does not increase under LOPC in the sense that E sq ( A ; B ) ρ ≥ E sq ( A ; B ) σ if Alice and Bob can obtain the state σ AB from ρ AB by LOPC [24] , [23] . The method for doing so was to exploit the fact that LOPC distillation of the secret key is equivalent to LOCC distillation of private states [30] , [31] . A private state has the following form [30] , [31] : where is a global unitary operation, is a maximally entangled state of Schmidt rank d and {| i › A } and {| i › B } are complete orthonormal bases for quantum systems A and B , respectively. Furthermore, the squashed entanglement is normalized, in the sense that E sq ( A ; B ) γ ≥log d (see Proposition 4.19 of ref. 24 ). Finally, the squashed entanglement satisfies the following continuity inequality [24] , [28] : if ‖ ρ AB − σ AB ‖ 1 ≤ ε , then where d ′=min{| A |,| B |} and h 2 ( x ) is the binary entropy function with the property that lim x →0 h 2 ( x )=0. The most general ( n , R , ε ) protocol in this setting is described as follows, where n is the number of channel uses, R is the key generation rate (measured in secret key bits per channel use) and ε is a parameter quantifying the security (see below for their formal definitions). The protocol begins with Alice preparing a state on n +1 systems. She then transmits the system A 1 through one use of the channel , and considering its isometric extension , we write the output state as . Let R (1) be a system that purifies this state. There is then a round of an arbitrary amount of LOPC between Alice and Bob, resulting in a state . This procedure continues, with Alice transmitting system A 2 through the channel, leading to a state , and so on. After the n th channel use, the state is (note that the dimension of the system A might change throughout the protocol). Let R ( n ) be a reference system that purifies this state. There is a final round of LOPC, producing a state , whose reduction ω AB satisfies where γ AB is a private state of nR bits. Note that we are implicitly including the systems A ′ and B ′ in A and B , respectively. We can now proceed by bounding the secret key generation rate of any such protocol as follows: The first inequality follows from the normalization of the squashed entanglement on private states (as mentioned above). The second inequality follows from the continuity of squashed entanglement, with an appropriate choice of f ( ε ) so that lim ε →0 f ( ε )=0 (see the Methods section for more details). To continue, we introduce the following new subadditivity inequality for the squashed entanglement: Lemma 2: For any five-party pure state , Proof: see the Supplementary Note 1 for a proof. With this new inequality in hand, we can establish the following chain of inequalities: The first inequality follows from monotonicity of the squashed entanglement under LOCC. The second inequality is an application of the subadditivity inequality in Lemma 2. The third inequality follows because (there is a particular input to the n th channel, while the systems AB 1 E 1 ⋯ B n −1 E n −1 R ( n ) purify the system being input to the channel). The sole equality follows because the squashed entanglement is invariant under local isometries (the isometry here being the isometric extension of the channel). The last inequality follows by induction, that is, repeating this procedure by using secrecy monotonicity and subadditivity, ‘peeling off’ one term at a time. Putting everything together, we arrive at which we can divide by n and take the limit as ε →0 to recover the result that P 2 ( )≤ E sq ( ). This completes the proof of Theorem 1. It should be stressed that the right hand of equation (4) is a ‘single-letter’ expression, meaning that the expression is a function of a single channel use. This is in spite of the fact that the quantity serves as an upper bound on the secret key agreement capacity, which involves using the channel many independent times, entangled input states, and/or measurements over many channel outputs. Lemma 2 is critical for establishing the ‘single letterization.’ The simple expression in equation (4) allows us to apply the bound to various channels, including the optical channel as shown below. In addition, as mentioned in the introduction, Theorem 1 states that E sq ( ) is a weak converse upper bound that bounds the key rate in the asymptotic limit of many channel uses. However, our bound is also valid for any finite number of channel uses, in the sense that the key rate is upper bounded in terms of E sq ( ) and the reliability and security of the protocol. It might be possible to improve upon our upper bound, by establishing a so-called strong converse theorem (see, for example, refs 32 , 33 ) or a refined second-order analysis, along the lines of ref. 34 , which is left as an important open question. We point the reader to the Methods section for a quantitative discussion and an example scenario involving a pure-loss optical channel. A variation of this setting is one in which there is a forward quantum channel from Alice to Bob and a backward quantum channel from Bob to Alice. The most general protocol for generating a shared secret will have Alice and Bob each prepare a state on n systems, Alice sending one system through the forward channel, them conducting a round of LOPC, Bob sending one of his systems through the backward channel, them conducting a round of LOPC, and so on. Using essentially the same proof technique as above, it follows that E sq ( )+ E sq () serves as an upper bound on the total rate at which Alice and Bob can generate a shared secret key using these two channels many independent times. It is also worth noting that E sq ( ) is an upper bound on the two-way-assisted quantum capacity Q 2 ( ) (defined in ref. 35 ) because P 2 ( )≥ Q 2 ( ) holds in general. Pure-loss optical channel Now we are in a position to derive a limit on the key generation rate of any QKD protocol that uses a lossy optical channel. The following input–output relation models linear loss in the propagation of an optical mode, such as through a lossy fibre or free space: where â , and ê are bosonic mode operators corresponding to the sender Alice’s input, the receiver Bob’s output and the environmental input, respectively. For the pure-loss bosonic channel, the environment mode is in its vacuum state. The transmittance of the channel, η ε[0,1], is the fraction of input photons that makes it to the output on average. Let η denote the channel from Alice to Bob. For a secret key agreement protocol assisted by two-way classical-communication over this channel, we assume that it begins and ends with finite-dimensional states; however, the processing between the first and final steps can be conducted with infinite-dimensional systems (see the Methods section for further discussion of this point). Furthermore, as is common in bosonic channel analyses [36] , we begin by imposing a mean input power constraint. That is, for each input mode, we require that ‹ â † â ›≤ N S , with 0≤ N S <∞. Thus, E sq ( η ), with the additional photon number constraint on the channel input is an upper bound on P 2 ( η ). By taking the squashing channel for the environment Eve to be another pure-loss bosonic channel of transmittance η 1 ε[0,1] (see Fig. 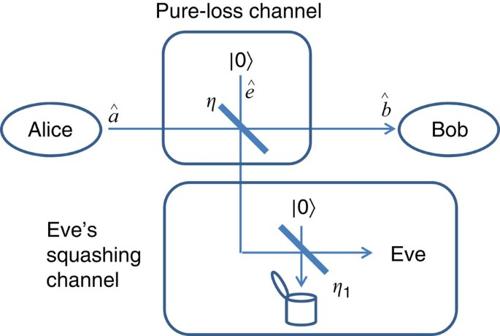Figure 2: Set-up for calculating the upper bound on the secret key rate of the pure-loss optical channel. Alice and Bob use a pure-loss optical channel with transmittanceηas their quantum channel. Eve holds the reflectance from the channel and applies her squashing channel constructed by a pure-loss optical channel with transmittanceη1. 2 ), noting that the resulting conditional mutual information can be written as a sum of two conditional entropies, and applying the extremality of Gaussian states with respect to conditional entropies [37] , [38] , we find that the following quantity serves as an upper bound on E sq ( η ) for all η 1 ε[0,1] (see Supplementary Note 2 for a detailed proof): Figure 2: Set-up for calculating the upper bound on the secret key rate of the pure-loss optical channel. Alice and Bob use a pure-loss optical channel with transmittance η as their quantum channel. Eve holds the reflectance from the channel and applies her squashing channel constructed by a pure-loss optical channel with transmittance η 1 . Full size image where g ( x )≡( x +1) log 2 ( x +1)− x log 2 x is the Shannon entropy of a geometric distribution with mean x . The function g ( x ) is also equal to the von Neumann entropy of a zero-mean circularly symmetric thermal state with mean photon number x . Since the function in (6) is symmetric and convex in η 1 , its minimum occurs at η 1 =1/2, leading to the following simpler upper bound: By taking the limit of this upper bound as N S →∞, we obtain the photon-number-independent expression, which recovers the upper bound stated in equation (1). As mentioned in the introduction, any excess noise in the channel can only reduce the squashed entanglement of a quantum channel, and thus equation (1) serves as a fundamental upper limit on the secret key agreement capacity of a lossy optical channel. This statement follows from a quantum data-processing argument, that is, the quantum conditional mutual information does not increase under processing (including noise additions) of one of the systems that is not the conditioning system (see Proposition 3 of ref. 22 ). Note that the statement does not prohibit the improvement of the key rates by applying ‘noisy processing’ in specific existing QKD protocols such as BB84 as proposed in refs 39 , 40 . However, such an improved key rate is always equal or lower than our bound in equation (1). It is instructive to compare our upper bound with the known lower bounds on the secret key agreement capacity of optical QKD protocols. BB84 is the most widely examined QKD protocol. When operating under polarization encoding and ideal conditions over a lossy channel (perfect single photon sources and detectors, and with the efficient BB84 protocol as proposed in ref. 41 ), and with no excess noise (that is, Eve can do only passive attacks consistent with the channel loss alone), the key rate is simply given by η /2 secret key bits per mode [2] , [41] . The best-known lower bound on the secret key agreement capacity of the pure-loss channel η was established in ref. 42 : These lower bounds and our upper bound are compared in Fig. 3 , where we also plot the rate achievable with coherent-state continuous variable protocol (CV-GG02) [2] , [9] , another major protocol, without any excess noise or imperfections. In addition, as examples of the practical performance of QKD, we plot the decoy-state BB84 protocol including device imperfections as well as the imperfect CV-GG02 with uncalibrated- and calibrated-device scenarios (see the Methods section for the details of the protocols and parameters). 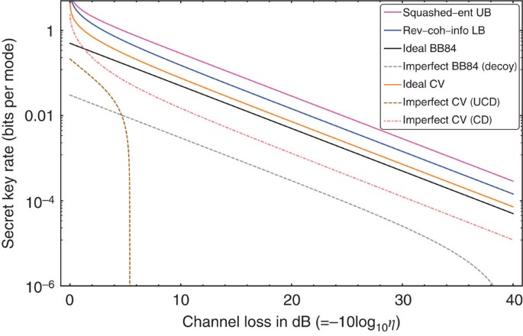Figure 3: Upper and lower bounds onP2for a pure-loss bosonic channel. The magenta solid curve is the squashed entanglement upper bound in equation (1). The blue solid curve is the reverse coherent information lower bound. The black solid curve is the efficient BB84 protocol with perfect devices and single photons, and the grey dotted curve is the decoy BB84 protocol including experimental imperfections2. The orange solid curve is the Gaussian modulated coherent-state continuous variable protocol (CV-GG02)9with perfect devices. The brown dashed and pink dash-dotted curves are the CV-GG02 protocols including experimental imperfections with the uncalibrated- and calibrated-device scenarios, respectively. The details of the protocols and device parameters are described in the Methods section. Figure 3: Upper and lower bounds on P 2 for a pure-loss bosonic channel. The magenta solid curve is the squashed entanglement upper bound in equation (1). The blue solid curve is the reverse coherent information lower bound. The black solid curve is the efficient BB84 protocol with perfect devices and single photons, and the grey dotted curve is the decoy BB84 protocol including experimental imperfections [2] . The orange solid curve is the Gaussian modulated coherent-state continuous variable protocol (CV-GG02) [9] with perfect devices. The brown dashed and pink dash-dotted curves are the CV-GG02 protocols including experimental imperfections with the uncalibrated- and calibrated-device scenarios, respectively. The details of the protocols and device parameters are described in the Methods section. Full size image We note the following important observations. First, the two bounds in equations (1) and (7) become close for η ≪ 1 (the high-loss regime, relevant for long-distance QKD). Thus, for small η , our upper bound demonstrates that the protocol from ref. 42 achieving the lower bound in equation (7) is nearly optimal. To be precise, the upper and the lower bounds are well approximated by 2 η /ln 2 and η /ln 2 key bits per mode, when η ≪ 1 (see Fig. 3 ). Furthermore, the ideal BB84 rate ( η key bits per mode) is worse than the reverse coherent information lower bound, only by a constant (2/ln 2≈2.88) factor in the high-loss regime where the factor 2 reflects the fact that the BB84 uses two polarization (or other) modes to send one bit, and ln 2 reflects some kind of gap between the qubit and continuous variable protocols. On the other hand, the protocol described in ref. 42 that attains the reverse coherent information rate requires an ideal SPDC source, and collective quantum operations and measurements, structured realizations of which are not known. In addition, even with detector impairments, both the decoy-state BB84 as well as the CV-GG02 protocol (with or without the assumption of calibrated devices) can achieve secret key rates that scale linearly with the channel transmittance, until a maximum channel loss threshold where the rate plummets to zero. For BB84, this loss value where the rate cliff occurs is driven by the detector dark counts, whereas for CV-GG02, it is driven primarily by the electronic noise in Bob's homodyne detector. Hence, given the comparisons shown in Fig. 3 , and since BB84 and CV protocols are realizable with currently available resources, it does not seem very worthwhile to pursue alternative repeater-less QKD protocols for higher key generation rate over a lossy channel. Second, our bound significantly advances one of the long-standing open problems in quantum information theory, that of finding a good upper bound on P 2 ( ), as well as for the two-way assisted quantum capacity Q 2 ( ) (number of qubits that can be sent perfectly per use of a quantum channel with two-way classical-communication assistance). This is true for a general quantum channel and, in particular, for optical quantum channels such as η . One of the important open questions is whether or not the true P 2 ( η ) is additive. In other words, the question is whether the protocol that attains P 2 ( η ) requires an input state that is entangled over several channel uses, or if a product input state suffices. In general, it is likely that P 2 ( ) is super-additive for some channels as is the case for the unassisted secret key agreement capacity P ( ) [43] and the classical capacity of quantum channels [44] . On the other hand, it is known that the classical capacity and the unassisted quantum capacity of the lossy optical (bosonic) channel are additive [36] , [45] . As mentioned above, our upper bound on P 2 ( ) is a single-letter expression for any channel, that is, the input optimization to evaluate our upper bound needs to be performed over a single channel use. The lower bound equation (7) is the single-letter reverse coherent information evaluated for the lossy bosonic channel, whose operational interpretation is an entanglement distribution rate achievable via a product input realizable using a two-mode squeezed vacuum state, and collective quantum operations in the subsequent steps of the protocol, which uses classical feedback [14] . Thus, despite the fact that the additivity question for P 2 ( η ) remains open, any super-additive gain cannot be very large in the high-loss regime, and P 2 ( η ) must scale as ~ η , when η ≪ 1. As a final point, consider a two-way QKD protocol, that is, when Alice and Bob may use the lossy optical channel η in both directions, and also communicate freely over a two-way public channel. In such a case, the secret key agreement capacity is upper-bounded by 2 log 2 ((1+ η )/(1− η )) secret key bits per mode transmitted in both directions. In summary, we have established in equation (1) an upper bound on the rate at which any QKD protocol can generate a shared secret key over a point-to-point lossy optical channel. This upper bound is a function of the channel loss only, and it does not increase with increasing transmit power. We compared our upper bound with the best-known lower bound on the key rate and a key rate attainable in principle by the BB84 and CV-GG02 protocols under ideal operating conditions. This comparison reveals that there is essentially no scaling gap between the rates of known protocols and the ultimate secret key agreement capacity, and thereby that there is no escaping the fundamental exponential decay of the key rate with distance. The result of this paper on one hand provides a powerful new tool for upper-bounding the private capacity with two-way classical communication assistance, for a general quantum channel. On the other hand, the application to QKD over optical channels strongly suggests the need for quantum repeaters to perform QKD at high rates over long distances, no matter which actual QKD protocol one may choose to use. Some important open questions remain. Although our bound applies for any finite number of channel uses, one might be able to improve upon our result by establishing a strong converse theorem or even better by considering a second-order analysis, along the lines discussed in ref. 34 . For establishing a strong converse theorem, some combinations of the ideas presented in refs 46 , 47 might be helpful. Another important open question is whether our upper bound in equation (1) could be achievable using some QKD protocols, or whether the bound can be further tightened by choosing a squashing channel for Eve other than the pure-loss channel (as shown in Fig. 2 ) or by investigating upper bounds other than E sq ( ). For this last question, some recent results in classical information theory [48] , [49] might be helpful. Weak converse Although our main result establishes only a weak converse theorem, it is possible to estimate the effect of a finite number of channel uses, which is always the case in any practical setting. We carefully estimate f ( ε ) discussed in the proof of Theorem 1. From the continuity inequality in (5), we can explicitly describe the additional term f ( ε ): where d =2 nR . This implies the following bound: In the limit of large n , the second term vanishes and the upper bound becomes which suggests that there might be room for a tradeoff between communication rate and error probability/security as quantified by ε . If one could establish a strong converse theorem, this would eliminate the implied tradeoff given above, in the ideal case showing that the bound R ≤ E sq ( ) would hold in the large n limit regardless of the value of ε . Let us consider a quantitative example, consisting of a pure-loss channel with ε =10 −10 and n =10 4 (these are not too far from realistic QKD parameters [4] ). For these values, we get Furthermore, a 200-km fibre with 0.2 dB km −1 corresponds to η =10 −4 and log((1+ η )/(1− η ))≈2.885 × 10 −4 . Replacing E sq ( ) with our upper-bound log((1+ η )/(1− η )) (see equation (1)) and plugging in the above values of ε and n , we find that which is rather close to log((1+ η )/(1− η ))≈2.885 × 10 −4 . However, one can improve upon our upper bound by establishing a strong converse theorem or even better by providing a refined second-order analysis along the lines discussed in ref. 34 . Infinite-dimensional system An optical channel can transmit infinite-dimensional (that is, continuous variable) quantum states, while Theorem 1 implicitly assumes finite-dimensional systems. We can circumvent this subtlety by assuming the protocol between Alice and Bob begins and ends with finite-dimensional states; however, the processing between the first and final steps can be conducted with infinite-dimensional systems. That is, their objective is to generate a maximally entangled state |Φ› AB or a finite number of secret key bits, and they do so by Alice encoding a finite-dimensional quantum state into an infinite-dimensional system and the final step of the protocol has them truncate their systems to be of finite dimension. In this way, the continuity inequality in the proof of Theorem 1 safely applies and all of the other steps in between involve only the quantum data-processing inequality, which has been proven to hold in the general infinite-dimensional setting [50] . Decoy-state BB84 and CV-GG02 protocols with experimental imperfections The asymptotic secret key rates of the decoy-state BB84 protocol and the CV-GG02 in Fig. 3 are calculated from the theoretical models including imperfections summarized in ref. 2 . The parameters used for the plots are as follows: for the decoy BB84, the visibility of interference at Bob’s receiver is 0.99, the transmittance of Bob’s device is unity, the detector efficiency is 0.2, dark count rate is 10 −6 and the information leakage parameter because of the practical error code is set to be 1.2. For the CV-GG02 protocol, the optical noise is 0.005, the detector efficiency is 0.5, the electronic noise of the detector is 0.01 and the efficiency of the error correction code is set to be 0.9. These parameters are chosen to reflect the state of the art device technologies. In the ‘uncalibrated-device’ scenario, Eve is able to access Bob’s homodyne detector imperfections, for example, to entangle the loss and noise of the detector. The ‘calibrated-device’ scenario is based on the assumption that the homodyne detector is calibrated in a secure laboratory such that Eve cannot entangle her system to the detector imperfections. This assumption allows Alice and Bob to significantly extend the key rate and the loss tolerance. Note that the purpose of these plots is to compare these protocols under imperfections with our fundamental upper bound but is not to compare the practical aspects between these protocols (for example, our model does not include important practical conditions such as phase stability, repetition rate of the system, actual coding strategies, and so on). For completeness, the key rate formulae for each protocol and scenario are described in Supplementary Note 3 . How to cite this article : Takeoka M., et al. Fundamental rate-loss tradeoff for optical quantum key distribution. Nat. Commun. 5:5235 doi: 10.1038/ncomms6235 (2014).